Morphological and population genomic evidence that human faces have evolved to signal individual identity Facial recognition plays a key role in human interactions, and there has been great interest in understanding the evolution of human abilities for individual recognition and tracking social relationships. Individual recognition requires sufficient cognitive abilities and phenotypic diversity within a population for discrimination to be possible. Despite the importance of facial recognition in humans, the evolution of facial identity has received little attention. Here we demonstrate that faces evolved to signal individual identity under negative frequency-dependent selection. Faces show elevated phenotypic variation and lower between-trait correlations compared with other traits. Regions surrounding face-associated single nucleotide polymorphisms show elevated diversity consistent with frequency-dependent selection. Genetic variation maintained by identity signalling tends to be shared across populations and, for some loci, predates the origin of Homo sapiens . Studies of human social evolution tend to emphasize cognitive adaptations, but we show that social evolution has shaped patterns of human phenotypic and genetic diversity as well. Human societies are predicated on our abilities to individually recognize and track scores of people in our social networks [1] , [2] . The complexity of human societies is widely recognized as a major selective force that has shaped our cognitive abilities and social intelligence [3] , [4] , [5] . Indeed, humans have highly developed individual recognition abilities, and there is a rich literature examining social cognition and individual recognition in humans [6] , [7] , [8] , [9] . In particular, facial recognition plays a critical role in human social interactions, and the cognitive mechanisms underlying facial recognition have been well studied [9] , [10] , [11] . When it comes to recognition, however, cognition is only one half of the equation. Recognition also depends on phenotypic variation in a population [12] , without which discrimination is impossible. Compared with other animals or other parts of our bodies, we perceive human faces as being unusually variable and easy to recognize ( Fig. 1 ). While this phenomenon can be at least partly explained by our specialization for learning human faces [10] , the fact that facial recognition is so important for social interactions among humans suggests that selection may have lead to increased facial distinctiveness. Despite the striking differences among human faces and the importance of facial identity for human society, the evolution of individuality in human faces has yet to be explored. 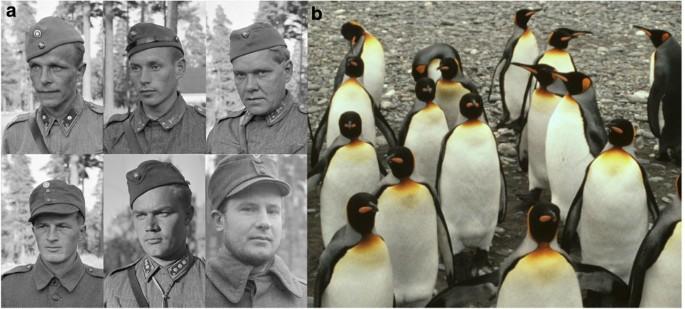Figure 1: Humans have much more individually distinctive faces than many animals. (a) Human populations show extensive variability in facial morphology that is used for individual recognition. Patterns of elevated variability are even maintained in more genetically homogeneous populations such as the Finnish, as demonstrated by the portraits of six male soldiers. (b) In contrast to the variability present in human faces, many animals such as king penguins have much more uniform appearances. While king penguins are not known to visually recognize individuals, they do have highly distinctive vocalizations that are used for individual recognition. (Photo credits: SA-kuva, Finnish Armed Forces photograph; Wikimedia commons.) Figure 1: Humans have much more individually distinctive faces than many animals. ( a ) Human populations show extensive variability in facial morphology that is used for individual recognition. Patterns of elevated variability are even maintained in more genetically homogeneous populations such as the Finnish, as demonstrated by the portraits of six male soldiers. ( b ) In contrast to the variability present in human faces, many animals such as king penguins have much more uniform appearances. While king penguins are not known to visually recognize individuals, they do have highly distinctive vocalizations that are used for individual recognition. (Photo credits: SA-kuva, Finnish Armed Forces photograph; Wikimedia commons.) Full size image Theoretical and empirical studies have proposed multiple non-mutually exclusive negative frequency-dependent selection (NFDS) pressures that may maintain elevated phenotypic diversity in natural populations. These include apostatic selection, in which predation is lower on rare prey [13] , [14] , mating preferences for novel phenotypes [15] and selection to be recognizable [16] . For example, both apostatic selection and frequency-dependent mate preferences have been shown to contribute to the maintenance of the highly variable and heritable male colouration patterns in the guppy ( Poecilla reticulata ) [14] , [17] . Frequency-dependent attractiveness has been proposed as a mechanism to explain patterns of hair and eye colour diversity in Europeans [18] and recent tests have found empirical support for frequency-dependent attractiveness of beards in human males [19] . Although elevated variation in guppy colouration is limited to adult males [17] , human facial individuality is not limited to a particular age or sex class, suggesting that frequency-dependent mate preferences are unlikely to be the sole or major driver of elevated diversity in human facial patterns. Indeed, individual recognition is important in humans from cradle to grave across multiple contexts. Selection to be individually recognizable in a variety of scenarios is therefore a prime hypothesis to explain the high diversity in human facial appearance [12] . Individual recognition will only evolve when it is beneficial to identify other individuals [12] . Whether or not individuals benefit by being identifiable and easily recognized raises a different question. Traits used for individual recognition are expected to evolve as either identity cues or as identity signals depending on the benefits of being recognized [12] , [20] , [21] . Identity cues are traits that allow discrimination but have not evolved for the purpose of recognition [22] and are not expected to show signatures of adaptive evolution. Cues are essentially inadvertent phenotypic variation that other individuals can use for discrimination [23] , [24] . For example, today human fingerprints are used for forensic identification though they have not evolved to facilitate recognition. As is the case for fingerprints, identity cues do not necessarily benefit individuals that are being recognized and may in fact harm them. In contrast, identity signals are traits that have been selected to facilitate individual recognition and as a result show elevated variation within populations [16] , [25] . Individual recognition can rely on cues alone, but if individuals benefit on average from being recognized then selection is expected to favour individuals to advertise their identity with distinctive phenotypes [12] , [20] , [21] . Identity signals evolve when being confused with others is costly due to misdirected behaviours including aggression [26] , mating opportunities [27] , parental care [28] and so on. Comparative and experimental evidence for identity signalling leading to increased phenotypic diversity has been documented in multiple taxa [25] , [26] , [28] , [29] but has not been investigated in humans. Individual recognition is facilitated when individuals display divergent trait values and novel combinations of traits [11] , [21] leading to disruptive selection on multiple traits and the evolution of independent developmental pathways [21] , [26] . Three key predictions of the identity-signalling hypothesis are (i) facial characteristics should be more variable than other visible traits not used for recognition, (ii) face traits are expected to show lower inter-trait correlations compared with other morphological traits and (iii) loci underlying normal facial variation are expected to show elevated genetic diversity consistent with NFDS favouring rare phenotypes. Loci contributing to identity-signalling traits are expected to show evidence of NFDS, such as an excess of intermediate-frequency alleles and elevated diversity when controlling for divergence [30] , [31] . Selection for identity signalling on any one facial trait is likely to be relatively weak as there are numerous traits that contribute to individual identity. Due to the complex genetic architecture of facial variation [32] , [33] , [34] , we expect a modest signature of elevated diversity in genomic regions underlying identity signals as a whole [35] , [36] , though there may be stronger evidence for NFDS at a subset of loci. While it is plausible that identity cues could also show elevated phenotypic variation and reduced phenotypic correlations as a result of relaxed selection or stochastic developmental processes, the loci underlying identity cues are expected to evolve neutrally. Thus even a weak signature of NFDS, as may be expected for a complex quantitative trait such as facial identity, would reject the cue hypothesis and provide support for identity signalling. Consistent with the predictions of the identity-signalling hypothesis, we find elevated phenotypic variation and reduced levels of inter-trait correlations in human faces compared with non-facial morphology. Furthermore, we find population genomic support for the identity-signalling hypothesis. Loci associated with variation in normal facial morphology show elevated nucleotide diversity compared with loci associated with variation in height or presumably neutral, intergenic variation. The loci with the strongest evidence of selection tend to be shared across continents, suggesting that selection on at least some loci associated with identity signalling is likely to be old. Indeed, by comparing sequences of modern humans with those of Neanderthals and Denisovans, we demonstrate that variation at some loci associated with facial morphology predates the origin of the human species. While studies of human social evolution have tended to emphasize its effect on cognition, our results suggest that social evolution has also played an important role in shaping human morphology. Morphological evidence Morphological comparisons between faces and other traits are consistent with the predictions of identity signalling. We tested these predictions using data for 18 facial and 46 non-facial linear distance measures from the ANSUR anthropometric study of US army personnel [37] for females and males of African and European American ancestry, respectively ( Supplementary Tables 1 and 2 ). Linear distances between facial landmarks have higher coefficients of variation than linear measurements of body traits in every group ( Fig. 2a , Mann–Whitney U (MWU)-test, n =18 facial and 46 non-facial measures, P <0.03 for all comparisons). Without selection for uncoupled development, traits within individuals are generally correlated, as larger individuals tend to have larger traits [38] , [39] . However, facial traits show lower inter-trait correlation coefficients than body traits in all four groups as predicted by the identity-signalling hypothesis ( Fig. 2b , MWU-test, n =153 facial correlations and 1,035 non-facial correlations, P <0.001 for all comparisons). Indeed, the vast majority of the body measures are correlated (percentage of significant Pearson’s correlations between traits, African American females (AAF)=95.17%, African American males (AAM)=99.14%, European American females (EAF)=96.62%, European American males (EAM)=99.81%, n =1,035 pairwise comparisons), though many fewer facial traits are correlated with each other (AAF=63.4%, AAM=73.9%, EAF=47.1%, EAM=84.2%, n =153 pairwise comparisons, Z -ratio <−11 and P <0.002 for all comparisons). Uncorrelated values for face traits increase the diversity of facial phenotypes, facilitating recognition. For example, the breadth and length of hands are correlated ( Fig. 2c , r 2 =0.30, P <0.0001), though the breadth and length of noses are not ( Fig. 2d , r 2 =0.002, P =0.06). These results add to previous findings that humans have among the lowest craniofacial morphological integration among primates and mammals more broadly [40] . 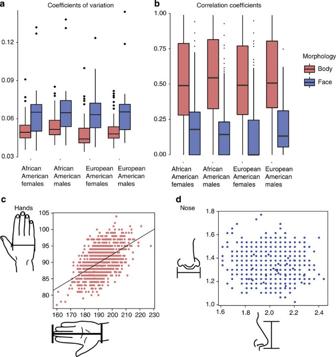Figure 2: Morphological evidence that human faces have evolved to signal individual identity. Morphological comparisons of facial features with other aspects of body morphology are consistent with selection for identity signals. (a) In all four groups examined, facial traits have higher coefficients of variation than other body traits (P<0.03 for all comparison). (b) Facial traits as a group show lower inter-trait correlations than non-facial traits in all four populations examined (P<0.001 for all comparisons). (c) For most traits, such as hands, larger individuals have larger traits such that the width and length of an individual’s hand are correlated. (d) In contrast to hands, the width and length of the nose are not correlated. Box plots show median and 25th and 75th percentiles (N=181 African American females; 457 African American males; 204 European American females; 1,168 European American males). TheP-values shown in the figure legend are from one-tailed Mamm-WhitenyUtests. The scatterplots show the trait values for European American male service members measured in the ANSUR II data set. Best-fit lines are shown for significant regressions. Figure 2: Morphological evidence that human faces have evolved to signal individual identity. Morphological comparisons of facial features with other aspects of body morphology are consistent with selection for identity signals. ( a ) In all four groups examined, facial traits have higher coefficients of variation than other body traits ( P <0.03 for all comparison). ( b ) Facial traits as a group show lower inter-trait correlations than non-facial traits in all four populations examined ( P <0.001 for all comparisons). ( c ) For most traits, such as hands, larger individuals have larger traits such that the width and length of an individual’s hand are correlated. ( d ) In contrast to hands, the width and length of the nose are not correlated. Box plots show median and 25th and 75th percentiles ( N =181 African American females; 457 African American males; 204 European American females; 1,168 European American males). The P -values shown in the figure legend are from one-tailed Mamm-Whiteny U tests. The scatterplots show the trait values for European American male service members measured in the ANSUR II data set. Best-fit lines are shown for significant regressions. Full size image Population genomic evidence Using data from the 1000 Genomes Project [41] , we tested for a signature of NFDS in genomic regions surrounding single nucleotide polymorphisms (SNPs) previously associated with differences in normal facial morphology in Europeans [32] , [33] . We compared the distribution of population genetic summary statistics calculated around face SNPs with the distribution of summary statistics for 5,000 putatively neutral intergenic regions as identified by the Neutral Region Explorer [42] . Here we present an analysis based on 2-kb windows, though the patterns of diversity reported here are robust to a range of window sizes ( Supplementary Fig. 1 ). Elevated diversity in face regions relative to the intergenic regions would be consistent with the predictions of NFDS. However, it is possible that morphological traits in general could show elevated diversity in comparison with neutral regions, so we also compared face regions with regions surrounding SNPs associated with height [43] , another complex morphological trait, as an additional control. Patterns of diversity surrounding face-associated SNPs are consistent with NFDS on complex quantitative traits as predicted under the identity-signalling hypothesis. Here we present the values for the Finnish population ( Fig. 3 ), though broadly similar overall patterns are found for other 1000 Genomes population samples from Europe and Africa and to a weaker extent Asia ( Supplementary Figs 2–9 ). The folded site frequency spectrum shows that regions surrounding face-associated SNPs have an excess of intermediate-frequency variants compared with the two sets of control loci ( Fig. 3a , MWU, P <0.0001 for both comparisons). Additionally, the distribution of summary statistics for faces differs from distributions found for height or intergenic regions consistent with NFDS on facial traits ( Fig. 3b–e , P <0.05 for all comparisons). One possible confounding factor is that intermediate-frequency SNPs are over-represented in genotyping panels [44] and thus more often associated with traits in genome-wide association studies, so elevated diversity could conceivably be confounded by ascertainment biases. Two lines of evidence argue against this. First, the association studies and population genomic analyses were conducted in different samples of Europeans, and the patterns of elevated diversity around face SNPs are also found in African and Asian populations. Second, in the Finnish examined here, the minor allele frequency of the focal SNPs is actually lower for faces than for height (MWU, P =0.028, Supplementary Fig. 10 ), suggesting that potential biases in association studies cannot explain the elevated patterns of diversity surrounding face-associated SNPs. The combination of elevated morphological and genetic diversity associated with human faces rejects a neutral explanation for human facial individuality and instead supports the hypothesis that human facial diversity is the product of selection for identity signalling in humans. 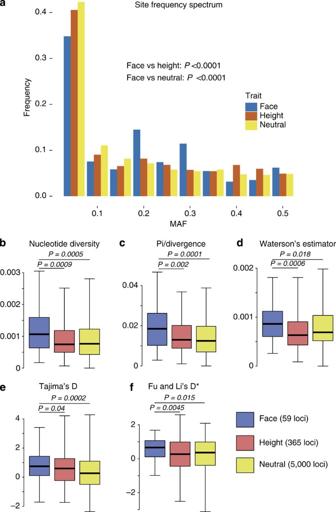Figure 3: Population genomic evidence that human faces have evolved to signal individual identity. Genomic regions associated with facial morphology show evidence of selection for identity signalling in the Finnish. (a) Face regions (N=59) have elevated levels of intermediate-frequency alleles compared with neutral regions (N=5,000) or genomic regions associated with variation in height (N=365). The bar graph shows the proportion of SNPs within each minor allele frequency (MAF) bin. (b) Additionally, face regions have elevated levels ofπ, (c) even after controlling for differing rates of divergence among loci. (d) Similarly, face regions show an elevated number of segregating sites, measured as Watterson’sθ. (e) Tajima’s D and (f) Fu and Li’s D* are elevated in facial regions compared to height and neural intergenic controls regions. Whiskers shows the 5th and 95th percentiles. Outliers are not shown so that the main distributions can be viewed at larger size. TheP-values shown are from one-tailed Mann–WhitneyU-tests. Note that sample sizes are reduced for tests corrected for divergence, as alignments were not available for all regions considered (N=58 face loci, 356 height loci, 4,873 neutral loci). Figure 3: Population genomic evidence that human faces have evolved to signal individual identity. Genomic regions associated with facial morphology show evidence of selection for identity signalling in the Finnish. ( a ) Face regions ( N =59) have elevated levels of intermediate-frequency alleles compared with neutral regions ( N =5,000) or genomic regions associated with variation in height ( N =365). The bar graph shows the proportion of SNPs within each minor allele frequency (MAF) bin. ( b ) Additionally, face regions have elevated levels of π , ( c ) even after controlling for differing rates of divergence among loci. ( d ) Similarly, face regions show an elevated number of segregating sites, measured as Watterson’s θ . ( e ) Tajima’s D and ( f ) Fu and Li’s D* are elevated in facial regions compared to height and neural intergenic controls regions. Whiskers shows the 5th and 95th percentiles. Outliers are not shown so that the main distributions can be viewed at larger size. The P -values shown are from one-tailed Mann–Whitney U -tests. Note that sample sizes are reduced for tests corrected for divergence, as alignments were not available for all regions considered ( N =58 face loci, 356 height loci, 4,873 neutral loci). Full size image Evolutionary dynamics of identity-signalling loci Due to the lack of data on SNPs associated with signalling traits in animals, population genomic methods have not previously been used to empirically explore the evolutionary dynamics of signalling traits. The present data set on identity signals in humans, however, provides an unprecedented opportunity to examine the history of selection on signalling traits used in social communication. Selection for identity signalling is expected to act on faces in all populations though it need not occur at the same loci. Conceivably, selection may act on the same loci across populations; different populations could maintain diversity at distinct loci underlying the same trait; or selection may act on loci underlying different traits in each population depending on the dynamics of selection as human populations expanded across the globe. We explored this question by assessing whether loci showing elevated diversity, where both π corrected for divergence with macaques and Tajima’s D both fall in the 95th percentile, were shared across populations. Indeed, a disproportionate number of loci show evidence of elevated diversity in at least one population for faces (9/58) compared with height (6/356; χ 2 =23.5, P <0.0001) and intergenic regions (57/4,873; χ 2 =78.8, P <0.0001, Fig. 4 ). Furthermore, the regions that show elevated diversity for faces are more consistent across continents than expected; five of nine regions show elevated diversity on at least two continents compared with 1 of 57 intergenic regions ( χ 2 =27.2, P <0.0002, Fig. 4 ). All nine regions identified as having elevated diversity in at least one population have high levels of π /divergence (>90th percentile) in both African populations examined here ( Supplementary Table S3 ). Additionally, analyses of the haplotype networks for the nine regions show greater allelic diversity in African populations, with European and Asian populations carrying a subset of the African haplotypes ( Supplementary Figs 11–19 ). These patterns of diversity and haplotype sharing across populations are consistent with an African origin of allelic variation at identity signalling loci predating human migration out of Africa. Population differentiation in facial morphology appears in part to be the result of differential loss of diversity in non-African populations, consistent with reduced morphological variation in populations with increased distance to Africa [45] . 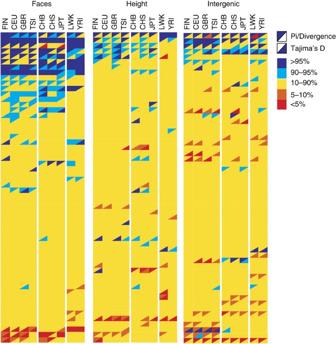Figure 4: Patterns of elevated diversity in face-associated loci across populations. The face-associated loci with elevated diversity consistent with selection for identity signalling tend to be shared across populations both within and between continents. The heatmap highlights loci on the extreme ends of the distributions forπ(controlling for divergence with macaque) and Tajima’s D. Columns correspond to populations and rows correspond to individual loci. Squares that are fully filled in with dark blue designate loci with evidence of elevated diversity (>95th percentile for both summary statistics). A greater number of loci show evidence of elevated diversity in at least one population for faces (9/58) compared with height (6/356;χ2=23.5,P<0.0001) and intergenic regions (57/4,873;χ2=78.8,P<0.0001). Additionally, patterns of elevated diversity are more consistently shared across populations for face-associated regions compared with the neutral regions (5/9 face regions versus 1/57 neutral regions,χ2=27.2,P<0.0002). To facilitate visual comparison, representative subsamples of height and intergenic regions are shown here. Subsamples were generated by randomly selecting loci from the height and neutral lists, which we confirmed did not deviate from the distribution of the total sample. All analyses reported were conducted on the full data sets. Figure 4: Patterns of elevated diversity in face-associated loci across populations. The face-associated loci with elevated diversity consistent with selection for identity signalling tend to be shared across populations both within and between continents. The heatmap highlights loci on the extreme ends of the distributions for π (controlling for divergence with macaque) and Tajima’s D. Columns correspond to populations and rows correspond to individual loci. Squares that are fully filled in with dark blue designate loci with evidence of elevated diversity (>95th percentile for both summary statistics). A greater number of loci show evidence of elevated diversity in at least one population for faces (9/58) compared with height (6/356; χ 2 =23.5, P <0.0001) and intergenic regions (57/4,873; χ 2 =78.8, P <0.0001). Additionally, patterns of elevated diversity are more consistently shared across populations for face-associated regions compared with the neutral regions (5/9 face regions versus 1/57 neutral regions, χ 2 =27.2, P <0.0002). To facilitate visual comparison, representative subsamples of height and intergenic regions are shown here. Subsamples were generated by randomly selecting loci from the height and neutral lists, which we confirmed did not deviate from the distribution of the total sample. All analyses reported were conducted on the full data sets. Full size image Here we present two examples highlighting the complex evolutionary trajectories of loci involved in identity signalling in humans. The examples illustrate (i) that genetic variation underlying identity signals tends to be old and of African origin and (ii) that phenotypic divergence between non-African populations is partly related to the differential loss of ancestral variation ( Fig. 5 ). Variants associated with the distance between the chin and bridge of the nose [33] are found within an intron of TMTC2 . A sliding window analysis of the region demonstrates that there is elevated diversity and reduced Fst consistent with sustained selection for identity signalling that is common to the three continental groups or occurred in their ancestral population ( Fig. 5a ). In contrast to the shared diversity at TMTC2 , intronic variants of SDK1 associated with nasal morphology [32] show a clear reduction of nucleotide diversity in Asian populations compared with the elevated diversity found in African populations. The reduction in diversity in Asian populations and increased Fst between Asian and African populations could either be the result of loss of diversity during population bottlenecks or directional selection on nasal morphology in Asian populations ( Fig. 5b ). For both loci, we constructed gene trees for the 5-kb window with the highest level of nucleotide diversity for 30 modern human sequences as well as the Neanderthal, Denisovan and chimpanzee sequences ( Fig. 5c,d ). Both trees provide further evidence for the ancient origins of loci under selection for identity signalling as archaic Hominin species are nested within modern human diversity. This result suggests that selection on some loci associated with identity signalling predates the origin of Homo sapiens and the emergence of modern facial morphology. 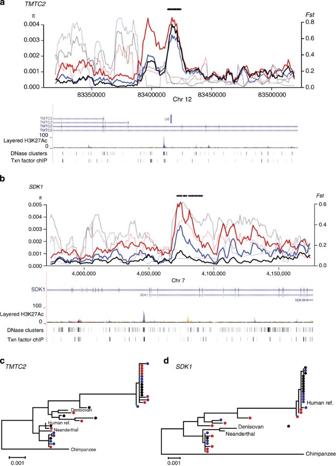Figure 5: Evolutionary history of example face-associated loci. Patterns of genetic diversity associated with facial morphology atTMTC2andSDK1. (a) AtTMTC2variation is largely shared across continents, while (b) atSDK1variation has been lost mainly in the CHB population. The sliding window analyses (a,b) show nucleotide diversity for three 1000 Genomes populations representing Europe (FIN), Asia (CHB) and Africa (YRI), respectively for 5-kb windows at 1-kb sliding intervals. Nucleotide diversity is shown with solid lines whileFstis represented by dotted lines. Colour of the lines represents the population examined forπ(FIN=blue, CHB=black, YRI=red) or the two populationFstcomparisons (FIN–YRI=red, CHB–YRI=black, FIN–CHB=blue) The locations of SNPs associated with facial morphology are shown as blue circles except for the focal SNP included in other window-based analyses that is denoted with a red circle. The UCSC Genome Browser tracks showing the locations of exons and three ENCODE regulatory regions, which show regions likely associated with genomic features involved in gene regulation, are shown below the sliding window. (c,d) Maximum likelihood trees show the relationships among 10 modern humans sampled from each of three populations (FIN, CHB and YRI) as well as sequences from Denisovan, Neanderthal and Chimpanzee. The modern human sequences are coloured according to their population of origin (FIN=blue, CHB=black, YRI=red). The region analyzed was the 5-kb window with the highest nucleotide diversity as determined by the sliding window analysis. Note that in both cases, the sequences for archaic Hominins are nested within modern human diversity, indicating the origin of the major haplogroups predates the evolution ofHomo sapiens. Figure 5: Evolutionary history of example face-associated loci. Patterns of genetic diversity associated with facial morphology at TMTC2 and SDK1 . ( a ) At TMTC2 variation is largely shared across continents, while ( b ) at SDK1 variation has been lost mainly in the CHB population. The sliding window analyses ( a , b ) show nucleotide diversity for three 1000 Genomes populations representing Europe (FIN), Asia (CHB) and Africa (YRI), respectively for 5-kb windows at 1-kb sliding intervals. Nucleotide diversity is shown with solid lines while Fst is represented by dotted lines. Colour of the lines represents the population examined for π (FIN=blue, CHB=black, YRI=red) or the two population Fst comparisons (FIN–YRI=red, CHB–YRI=black, FIN–CHB=blue) The locations of SNPs associated with facial morphology are shown as blue circles except for the focal SNP included in other window-based analyses that is denoted with a red circle. The UCSC Genome Browser tracks showing the locations of exons and three ENCODE regulatory regions, which show regions likely associated with genomic features involved in gene regulation, are shown below the sliding window. ( c , d ) Maximum likelihood trees show the relationships among 10 modern humans sampled from each of three populations (FIN, CHB and YRI) as well as sequences from Denisovan, Neanderthal and Chimpanzee. The modern human sequences are coloured according to their population of origin (FIN=blue, CHB=black, YRI=red). The region analyzed was the 5-kb window with the highest nucleotide diversity as determined by the sliding window analysis. Note that in both cases, the sequences for archaic Hominins are nested within modern human diversity, indicating the origin of the major haplogroups predates the evolution of Homo sapiens . Full size image Here we have presented both morphological and population genomic evidence consistent with the hypothesis that selection for individual identity signals has shaped patterns of human facial diversity. Though the evidence for selection at individual loci is modest, as expected for molecular evolution of polygenic traits [35] , the combination of morphological and genomic data from multiple populations clearly rejects the identity cue hypothesis and provides compelling evidence consistent with the idea that selection for individual identity signalling has shaped patterns of facial morphology in humans. Provided that the variation used in identity signals is not developmentally costly to produce or maintain, even a small selective advantage of individuality is expected to give rise to elevated phenotypic diversity when confusion is costly [21] . Previous studies have shown that being confused with others may be costly in a range of circumstances including within social hierarchies in Polistes wasps [26] , sexual selection in house mice [27] and parent–offspring interactions in cliff swallows [28] . It is unknown at present, which aspects of human sociality have been the most important sources of selection for identity signalling though it is likely that multiple facets of social interactions contribute to selection for identity signals. Individual recognition and discriminating among individuals plays a role in shaping important human behaviours including kin recognition [46] , investment in offspring [47] and cooperation [48] . It is likely that many social contexts favour identity signalling in humans, so it will be important for future research to explore the relative benefits of individuality across many social contexts and developmental stages in humans. In addition to selection for identity signalling, it is possible that other frequency-dependent process such as preferences for mates with rare or novel features could have played a role in shaping human diversity. For example, a recent study showed frequency-dependent effects on the attractiveness of male facial hair styles [19] . Preferences for individuals with rare phenotypes have also been shown in other animals, such as guppies where rare phenotypes confer a survival advantage due to reduced predation [14] , [17] . In humans, females tend to advertise physical attractiveness to mate more prominently than do males, who tend to advertise resources or performance ability [49] , [50] . Thus if frequency-dependent mate preferences were the major driver in determining facial identity, then females might be expected to show elevated levels of individuality compared with males just as female preferences for novel individuals contributes to the elevated colour pattern variation seen in male guppies [17] . However, in humans both males and females show elevated individuality in faces compared with other external morphology ( Fig. 2 ), suggesting that mate preferences alone cannot explain the patterns observed here. Similarly, mate preferences might be expected to drive variation only in adults as is observed in guppies [17] , yet distinctive facial morphology is seen at all life stages in humans. To the extent that frequency-dependent mate preferences play a role in shaping patterns of facial individuality, it is likely that mating preferences and identity signalling would have a positive feedback. If individual distinctiveness is beneficial in non-sexual contexts, preferences for mates with rare phenotypes may then also provide an additional benefit to distinctiveness [15] . Finally, our data do not preclude potential directional or stabilizing selection pressures that may arise from other potential mating preferences [51] or climate [52] on particular features of human facial morphology, though directional and stabilizing selection do not predict elevated genetic diversity within populations at the associated loci and so cannot explain the patterns of elevated genetic variation we have documented here. It is important to note that facial recognition is widespread in primates [53] and identity signalling is unlikely to be limited to human facial morphology, though the loci under selection may vary considerably across species. This may be especially true for humans, which have undergone considerable directional evolution of facial form during the course of hominin evolution [54] . While faces are a key feature used in human social recognition, other traits such as our voices also contribute to recognition and may have also experienced selection for identity signalling. Additionally, the strength of selection for particular identity-signalling traits may have changed over time in modern humans as cultural practices gave rise to individually distinctive clothing and hairstyles, which provide additional cues to identity. Traditional treatments of social selection in human evolution have emphasized the potential role for social interactions in shaping our cognitive abilities [3] , though our work demonstrates that social selection has shaped our morphology as well to facilitate social recognition. Importantly, our work draws a link between social interactions and the maintenance of genetic variation underlying traits used in social recognition. Social recognition is found across disparate animal taxa suggesting that selection for identity signalling is likely to be a common mechanisms generating phenotypic variation and maintaining genetic variation. Morphological analyses We examined morphological relationships among body parts and facial features using published anthropometric data sets. We focused our analyses on the ANSUR II data set because it provides a large, consistent database of individual level facial and body measurements. We analyzed the linear anthropometric measurements ( Supplementary Tables 1 and 2 ). In our analysis, we considered four groups of service members based on their sex and racial identity: African American females ( n =181, mean height=64.29±0.17 inches), African American males ( n =457, mean height=69.12±0.13 inches), European American females ( n =204, mean height=64.27±0.15 inches), and European American males ( n =1,168, mean height=69.32±0.08 inches). Compared with the general civilian population, the individuals measured in the ANSUR II data set tend to be taller and have lower levels of body fat [55] . Neither of these factors should influence our results or conclusions because our comparisons use facial and body measurements from the same individuals. Identity signalling predicts that traits used for recognition will have greater variance and be less correlated with each other compared with non-recognition traits in the same group of individuals. Using the ANSUR II data set, we tested two predictions of the identity-signalling hypothesis. First, we considered the levels of variation in each trait by calculating the coefficient of variation—by dividing the standard deviation of each trait by the mean. Coefficients of variation provide a scale-free method for comparing variation across samples that differ in average size as is the case for human morphological data. Second, we considered the correlations among traits by calculating the inter-trait Pearson’s correlations for all pairwise combination of traits within each class of traits. To compare the distribution of correlation coefficients between bodies and faces, we recorded the correlation coefficients significant at the P <0.05 level. For any pair of traits which did not show a significant correlation at P <0.05, we recorded the correlation as 0. Pearon’s correlation test is sensitive to the sample size such that correlations are more likely to be significant when larger samples are used. Therefore, comparisons between the different groups considered should be made with caution because of differences in sample size. For example, differences in the percentage of significant pairwise comparisons between males and females likely reflect differences in samples sizes. Within a group, however, the same individuals were measured for both facial and body traits, providing a direct comparison of the relative degree of correlation among traits. Selection of genomic regions for analysis Face-associated SNPs were taken from two recent genome-wide association studies of normal facial morphology. Paternoster et al. [33] conducted a discovery phase association study where they examined the relationship between facial characteristics and more than 2.5 million imputed SNPs in a sample of 2,185 15 year olds from the Avon Longitudinal Study of Parents and their Children [56] . Only subjects who genetically clustered with the CEU HapMap population were included in their analysis. The study identified 30 loci associated with facial morphology at P <5 × 10 −7 , which we examined in our study. Liu et al. [32] examined the relationship between facial morphology and more than 2.5 million SNPs in a discovery phase association study of 5,388 adults. The samples in the Liu et al. [32] study came individuals of European ancestry living in the Netherlands, Australia, Canada, Germany and the United Kingdom. They identified 29 loci associated with facial morphology at P <5 × 10 −7 , which we examined in this study. None of the SNPs identified by the two studies overlapped, providing a total of 59 loci for investigation. In both studies, multiple linked SNPs were often identified in association with a particular phenotype. When more than one SNP was associated with a trait, we chose the SNP with the smallest P -value within a 1-MB region of a chromosome from the association study. The SNPs identified for further examination from the two studies include one from each of 59 loci distributed throughout the autosomes. The SNPs are largely intergenic (95%) though a few occur within introns (5%). None were located in coding regions. We compared face-associated genomic regions with two sets of control regions. First, we examined SNPs associated with height taken from the genome-wide association study catalog of the National Human Genome Research Institute ( www.genome.gov ) on 25 April 2013. In order to prevent multiple sampling of any regions, we only considered SNPs that were separated by more than 4 kb. In the instances where multiple nearby SNPs had been associated with height, we chose the SNP that had been associated with the smallest P -value as reported in the genome-wide association study catalog. We excluded six SNPs associated with height that fall within the HLA region, though including the SNPs in our analyses does not alter our pattern of results. This produced a total of 365 loci associated with variation in height. Like faces, height is a composite character that depends on the morphology of numerous different bones. Additionally, both height and facial morphology have complex genetic bases with many loci of small effect contributing overall phenotypic variation [43] . SNPs associated with height are predominantly located in intronic regions (54%) and intergenic regions (36%) with a smaller percent found near the 3′ and 5′ end of genes (6%) or exons (3%). Second, we considered the genome-wide patterns of diversity by examining 5,000 2 kb intergenic regions. We identified putatively neutral intergenic regions in Europeans using the Neutral Region Explorer webserver [42] . The same set of intergenic regions was used for all populations. We analyzed regions surrounding the SNPs identified by the association studies at a set window size. The causative mutations underlying the traits are not known, though are likely to be located near the SNPs identified through genome-wide association studies [57] . The a priori best choice for a window size is not clear, though the patterns of elevated nucleotide diversity we observer are seen over a range of window sizes ( Supplementary Fig. 1 ). We chose to analyze 1 kb both up and downstream of the SNPs, providing windows of 2 kb. Smaller window sizes show marked increased variance in the summary statistics across loci ( Supplementary Fig. 1 ), though this variance levels off at window sizes of 2 kb or greater. Summary statistics We calculated summary statistics for each population using binary SNP and indel data from 1000 Genome Project Phase 1 variants. Nine non-admixed populations originating from Europe (CEU: Utah residents with Northern and Western European Ancestry; GBR: British from England and Scotland; FIN: Finnish from Finland; TSI: Toscani from Italia), Asia (CHB: Han Chinese in Beijing, China, CHS: Southern Han Chinese, JPT: Japanese from Tokyo, Japan) and Africa (LWK: Luhya from Webuye, Kenya; YRI: Yoruba from Ibadan, Nigeria) were considered in our study. We downloaded the population data to Galaxy [58] using the Table Browser function of the UCSC genome browser. We filtered the data based on the sets of 2-kb windows for face, height and intergenic regions to produce three files for each population, which we subsequently examined using custom macros in Excel. We used folded site frequency spectra to examine the distribution of minor allele frequencies among SNPs found within each of the demarcated regions. The expected distribution of allele frequencies at loci underlying a polygenic trait under negative frequency-dependent selection is unclear and will depend on the exact form of selection and the genetic architecture of the trait [59] . Nonetheless, frequency-dependent selection is expected to maintain alleles in a population, on average, longer than expected for neutral alleles [60] . Thus, the distribution of allele frequencies should differ from that expected in a stationary population at mutation drift equilibrium. In particular, we expect fewer rare alleles under a scenario of frequency-dependent selection. Spectra were compared using the raw counts of SNPs with each minor allele frequency using a MWU-test. To graph the folded site frequency spectra, we binned data into ranges of minor allele frequencies. In addition to the aggregated site frequency spectrum analysis, we also considered the distribution of multiple summary statistics of genetic diversity across the loci considered within our study. We calculated the following summary statistics for each 2-kb window: π , π corrected for human–macaque divergence, Watterson’s θ, Tajima’s D and Fu and Li’s D*. Both π and θ are estimators of the neutral mutation parameter, 4 N e μ. π is based on the number of pairwise differences among sequences within a sample and θ is based on the proportion of segregating sites. Loci under frequency-dependent selection are expected to show elevated values for π because frequency-dependent selection maintains alleles over longer periods of time. Older alleles accumulate mutations and therefore show higher levels of pairwise sequence divergence. We also examined the distribution of π corrected for the rate of divergence between humans and macaques. Different regions of the genome are known to experience differences in rates of mutation [61] . Loci with higher mutation rates will show elevated levels of π . The rate of divergence between humans and macaques provides a means of estimating the relative differences in mutation rates among loci [62] . The maintenance of multiple alleles in a population under frequency-dependent selection is also expected to lead to higher estimates of θ . Tajima’s D is the normalized difference between π and θ . Tajima’s D takes on positive values when there is an excess of intermediate-frequency variants and negative values when there is an excess of rare variants. Fu and Li’s D* is based on the number of nucleotide variants observed only once in a sample [63] . Negative measures of Fu and Li’s D* indicate an excess of singletons. Loci under frequency-dependent selection are expected to have a relatively smaller number of singletons and therefore more positive values of Fu and Li’s D*. We calculated the summary statistics using the allele frequencies given in the phase 1 variant files from the 1000 Genomes project. The short indels recorded in the data set were considered in the same manner as SNPs. Human–macaque divergence data were estimated using the LastZ alignment of the two reference genomes. Only regions with alignments between the two species’ genomes were considered in the analysis of π corrected for divergence with macaques (faces=58 regions, height=356 regions, neutral=4,873 regions) and for subsequent analyses using this statistic. For the aligned regions, the average alignment lengths were 1,832.21±4.49 sites out of 2,000. We compared the distribution of summary statistics for face-associated loci with the distributions for the two control data sets using one-tailed MWU-tests. Patterns of diversity across populations We asked whether the same loci showed elevated diversity in different populations. To do this, we identified loci in each population for which π /divergence and Tajima’s D were above the 95th percentile as determined from the empirical distribution of intergenic regions examined within that population. We then asked whether or not a disproportionate number of loci with elevated diversity was shared between continents for face regions compared with the intergenic regions examined. For the nine loci showing elevated diversity in at least one population, we investigated the patterns of haplotype sharing across populations. We examined the sequences in the 2-kb window used for previous analyses. For those coordinates, we downloaded a combined PED file including CHB, FIN and YRI from the 1000 Genomes project site (browser.1000genomes.org). We converted the PED files to fasta format using PGD Spider [64] . This procedure produced a fasta file containing the polymorphic sites found within the examined loci. Using the ‘pegas’ package in R [65] , we created haplotype networks for each of the loci. Sliding window analyses To examine the extent to which selection for identity signalling has been shared or divergent across continents, we conducted a sliding window analysis of the regions identified as having elevated diversity in at least one population. We calculated π and Fst for 5-kb windows every 1 kb for a total of 200 kb. π was calculated for one representative population for each continent (FIN, CHB and YRI). We estimated levels of differentiation between populations using Hudson’s Fst following ref. 66 as it produces unbiased estimates of Fst and is less sensitive to sample size and rare variants than other estimates of Fst such as Weir and Hill [67] . We estimated Fst for each set of SNPs considered by calculating a ratio of averages rather than an average of ratios, as the former is less sensitive to the presence of rare variants in a sample [66] . The SNPs identified in association with facial morphology are not found in coding sequences, so they are likely to influence gene regulation or splicing in some manner. For the two loci examined in greater detail, we used the UCSC genome browser to identify polymorphic sites in ENCODE regulatory regions. We focused on three ENCODE tracks in the UCSC browser [68] : H3K27Ac marks, DNase sensitivity clusters and transcription factor-binding sites. The H3K27Ac marks show regions for which there is CHIP-seq based evidence of enrichment for the H3K27Ac histone mark. H3K27 acetylation is associated with enhanced transcription. DNase sensitivity clusters show regions sensitive to DNase as assessed across 125 cell types. Promoters and other regulatory regions tend to be DNase sensitive. The transcription factor track shows regions with evidence of transcription factor-binding sites. Gene trees For the two 5-kb loci examined, we constructed maximum likelihood gene trees with 10 sequences each from the FIN, CHB and YRI 1000 Genomes populations for a total of thirty sequences. Additionally, we included the human and chimpanzee reference sequences as well as sequences for Denisovans [69] and Neanderthals ( http://cdna.eva.mpg.de/neandertal/altai/AltaiNeandertal/bam/ ). We downloaded the alignment of the human and chimpanzee reference sequences from Ensembl. Denisovan sequences were downloaded using the Table Browser function of the UCSC Genome Browser. The draft Altai Neaderthal sequences were downloaded for the relevant chromosomes from the Department of Evolutionary Genetics at the Max Planck Institute’s website. We constructed individual sequences for the 1000 Genomes, Denisovan and Neanderthal by manually altering the human reference sequence in accordance with the data found in the respective VCF files using Mega 5.2.1 (ref. 70) [70] . For the phased 1000 Genomes data, we selected one chromosome per individual sample. For the Neanderthal and Denisovan sequences, we included all of the sites that differed from the human reference to make a single sequence. After removing sites with gaps in the alignment, we constructed a maximum likelihood tree using a general time reversible model with a gamma distribution of invariant sites. How to cite this article: Sheehan, M. J. and Nachman, M. W. Morphological and population genomic evidence that human faces have evolved to signal individual identity. Nat. Commun. 5:4800 doi: 10.1038/ncomms5800 (2014).